Structural modelling and mutant cycle analysis predict pharmacoresponsiveness of a Nav1.7 mutant channel Sodium channel Na V 1.7 is critical for human pain signalling. Gain-of-function mutations produce pain syndromes including inherited erythromelalgia, which is usually resistant to pharmacotherapy, but carbamazepine normalizes activation of Na V 1.7-V400M mutant channels from a family with carbamazepine-responsive inherited erythromelalgia. Here we show that structural modelling and thermodynamic analysis predict pharmacoresponsiveness of another mutant channel (S241T) that is located 159 amino acids distant from V400M. Structural modelling reveals that Na v 1.7-S241T is ~2.4 Å apart from V400M in the folded channel, and thermodynamic analysis demonstrates energetic coupling of V400M and S241T during activation. Atomic proximity and energetic coupling are paralleled by pharmacological coupling, as carbamazepine (30 μM) depolarizes S214T activation, as previously reported for V400M. Pharmacoresponsiveness of S241T to carbamazepine was further evident at a cellular level, where carbamazepine normalized the hyperexcitability of dorsal root ganglion neurons expressing S241T. We suggest that this approach might identify variants that confer enhanced pharmacoresponsiveness on a variety of channels. Chronic pain affects more than one-quarter of Americans and pain in nearly 40% of these patients is not relieved by currently available drugs [1] . Recent studies have demonstrated that Na V 1.7, a voltage-gated sodium channel preferentially expressed in dorsal root ganglia (DRG) and sympathetic ganglia neurons, is essential for pain transduction [2] , [3] , [4] , [5] . Loss-of-function Na V 1.7 mutations cause congenital indifference to pain [6] , whereas gain-of-function mutations produce several painful syndromes including inherited erythromelalgia (IEM), a disorder in which, as a result of hyperpolarized activation of Na V 1.7, threshold is reduced and evoked firing frequency increased in pain-signalling DRG neurons, leading to intense burning pain [4] , [7] , [8] . These studies have validated Na V 1.7 as a molecular target for development of new pain therapeutics. IEM is characteristically unresponsive to existing pharmacotherapies [7] . Against this background of pharmaco-unresponsiveness, multiple-affected members of one family, carrying the Na V 1.7-V400M mutation, have responded favourably to carbamazepine (CBZ) [9] , a state-dependent sodium channel blocker used mainly for treatment of epilepsy and trigeminal neuralgia [10] . Our previous study demonstrated that therapeutic concentrations of CBZ normalize the hyperpolarizing shift of Na V 1.7-V400M mutant channel activation [9] , while not affecting activation of wild-type channels. As the shift of activation voltage dependence is a strong contributor to hyperexcitability of DRG neurons expressing IEM mutations [11] , normalization of activation in V400M by CBZ seems to underlie the beneficial effect of CBZ in this family [9] . These findings suggest the feasibility of personalized pharmacotherapy-based upon a pharmacogenomic approach. To achieve this goal, better understanding of structure–function relationships of human Na V 1.7 channel mutations that underlie drug responsiveness and development of pre-clinical assays of pharmacoresponsiveness are needed. The first demonstration of the crystal structure of an ion channel, KcsA [12] , provided a basis for structural modelling of the ion channel superfamily. Recently, the crystal structure of the bacterial voltage-gated sodium channel NavAb has been solved, shedding new light on structural substrates for channel gating and drug accessibility [13] . Starting from modelling of the human Na V 1.7 channel, we demonstrate in this study that an approach combining structural modelling, thermodynamic mutant cycle analysis and voltage- and current-clamp recording of Na V 1.7 mutant channels can predict pharmacoresponsiveness of a Na V 1.7 mutant channel (S241T) to CBZ, suggesting a novel approach to screening for amino-acid variants that enhance pharmacoresponsiveness of a variety of channels. V400 and S241 show atomic proximity in human Na V 1.7 channel Previous observations from the primary protein sequence suggest that IEM mutations of Na V 1.7 tend to cluster in transmembrane segments and S4–S5 linkers of domains I–III (ref. 4 ) but their proximity to each other within the folded structure is not clear. To better understand structure–function relationships among IEM mutations, we constructed a structural model of transmembrane helices of human Na V 1.7 channel based on the recently solved crystal structure of the bacterial voltage-gated sodium channel NavAb [13] . The human Na V 1.7 structural model was constructed using the GPCR-ITASSER program, an extension of the well-established I-TASSER algorithm [14] , [15] , incorporating a composite set of transmembrane-specific force fields and constraints [16] . Accuracy of individual domain models can be reliably estimated by the confidence score ( C -score), which has a high correlation to the actual TM-score [17] , a widely used measure of similarity between two protein structures with values in the [0,1] range. Unlike RMSD (root-mean-square-deviation) score, TM-score is insensitive to local structure variation and protein size. In general, two structures with TM-scores <0.17 correspond to random similarity and those with TM-scores >0.5 indicate high similarity between the predicted model and native structure [18] , [19] . Estimated TM-scores based on C -scores for our models of domains I–IV were 0.575, 0.805, 0.681 and 0.722, respectively, indicating similar folding structures to those of the bacterial sodium channel. The linear schematic of Na V 1.7 channel is shown in Fig. 1a . Assembled folded structural models are shown in Fig. 1b (intra-membrane side view) and Fig. 1c (cytosolic view). We are interested in the V400M mutation of DI/S6 helix because it is known to be pharmacoresponsive to CBZ [9] . Reasoning that location of V400M in the folded channel might be critical for its pharmacoresponsiveness, we looked for IEM mutations that are structurally close to V400M. Interestingly, our structural model revealed that the location of another IEM mutation (S241T) of DI/S4–S5 linker is close to that of V400M. The distance between S241 and V400 is only 2.4 Å measured from the closest hydrogen in the folded channel. This proximity, however, does not necessarily mean that the two residues engage in a direct interaction. Zoom-in views of DI/S6 show locations of V400 and S241 ( Fig. 1d ). The V400 side chain points toward the S4–S5 linker, where S241 is located ( Fig. 1d ). Although the effect of S241T on channel activation has been linked to increased size of the side chain at position 241 (probably through a steric hindrance effect) [20] , pharmacoresponsiveness of S241T mutant channel has not been previously assessed. 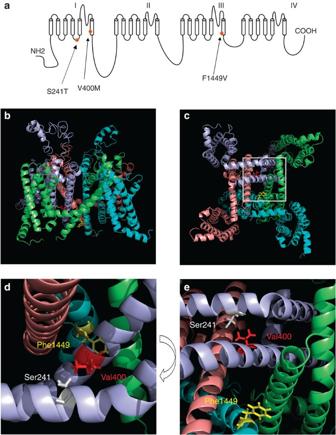Figure 1: Structural modelling of transmembrane domains of human NaV1.7 channel. (a) Schematic of the human NaV1.7 channel topology showing the mutations S241T, V400M and F1449V. (b) Intra-membrane view of structural model of NaV1.7 channel transmembrane domains. Domain I, light blue; Domain II, salmon; Domain III, cyan; Domain IV, lime. (c) Cyotsolic view of the structural model of NaV1.7 channel transmembrane domains. Boxed area containing S241, V400 and F1449 residues is enlarged in panele. (d) Close-up intra-membrane view of the area containing S241, V400 and F1449 residues. (e) Close-up cytosolic view of the boxed area of panelc. S241, V400 and F1449 are shown as stick and coloured grey, red and yellow, respectively. Figure 1: Structural modelling of transmembrane domains of human Na V 1.7 channel. ( a ) Schematic of the human Na V 1.7 channel topology showing the mutations S241T, V400M and F1449V. ( b ) Intra-membrane view of structural model of Na V 1.7 channel transmembrane domains. Domain I, light blue; Domain II, salmon; Domain III, cyan; Domain IV, lime. ( c ) Cyotsolic view of the structural model of Na V 1.7 channel transmembrane domains. Boxed area containing S241, V400 and F1449 residues is enlarged in panel e . ( d ) Close-up intra-membrane view of the area containing S241, V400 and F1449 residues. ( e ) Close-up cytosolic view of the boxed area of panel c . S241, V400 and F1449 are shown as stick and coloured grey, red and yellow, respectively. Full size image Another IEM mutation (F1449V) [21] was selected for analysis because it is located at the cytoplasmic end of S6 helix, which brings it into proximity with the V400M mutation in DI/S6 ( Fig. 1d ). Based on homology modelling to potassium channel structure, F1449 has been suggested to contribute to a hydrophobic ring at the cytoplasmic pore opening, which acts as an activation gate [22] . Modelling of F1449 using the bacterial sodium channel structure recapitulated the hydrophobic ring. However, like the S241T mutant, the pharmacoresponsiveness of F1449V mutant channel is unknown. V400M and S241T are energetically coupled during activation. Previous studies show that all of these IEM mutations hyperpolarize channel activation [4] , [9] , [20] , [21] , [22] . However, it is not clear whether these mutations work independently or in concert to affect the same or different aspect of activation. We therefore asked whether the location of Na V 1.7 channel mutations demonstrated by our structural modelling might indicate mechanistic coupling during channel activation. Thermodynamic mutant cycle analysis is a well-established approach for measuring independence or coupling of two mutations of a given protein [23] , [24] . We studied the coupling of V400M, a mutation located in the S6 helix, with either a structurally close mutation in the S4–S5 linker (S241T) or with a mutation in a different S6 helix (F1449V). Constructs carrying double mutations, for example, V400M and S241T or V400M and F1449V (named VM/ST and VM/FV, respectively) were created for mutant cycle analysis. Voltage dependence of activation was determined for Na V 1.7 WT channel, single mutations (V400M, F1449V and S241T) and double mutations (VM/ST and VM/FV) in transiently transfected HEK293 cells. If two mutations are energetically coupled (or affect channel activation through the same or shared mechanism), then the double mutation would not have an additive effect on channel activation compared with the single mutations. However, if two mutations are not energetically coupled (or affect the channel independently through distinct mechanisms), then the double mutation would have an additive effect on channel activation compared with the two single mutations. The voltage dependence of activation for WT, the mutant pairs to be evaluated and the corresponding double mutant were fitted with the Boltzmann equation to determine the V 1/2 (half-activation voltage) and Z (proportional to the slope at half activation)( Fig. 2a ). Representative traces are shown in Fig. 2c–h . Activation of double mutation VM/ST was rather close to that of the single mutations, indicating a non-additive effect and suggesting that V400M and S241T mutations alter activation via a common, shared mechanism ( Fig. 2a ). In contrast, activation of double mutation VM/FV was more hyperpolarized relative to the single mutations ( Fig. 2b ), indicating an additive effect and suggesting that the V400M and F1449V mutations alter activation via different, energetically independent mechanisms. 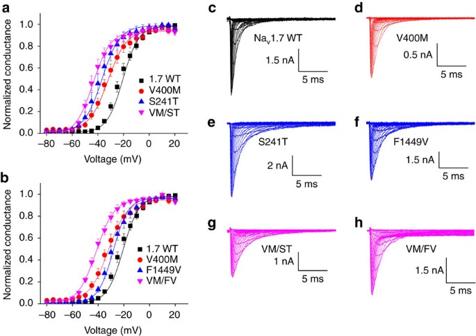Figure 2: Mutant cycle analysis of voltage dependence of activation of NaV1.7 mutations. (a) Voltage dependence of activation curves of NaV1.7 WT, V400M, S241T, and V400M/S214T (VM/ST) double mutant channels. Curves were Boltzmann fits of the data. (b) Voltage dependence of activation curves of NaV1.7 WT, V400M, F1449V and V400M/F1449V (VM/FV) double mutant channels. (c–h) Representative traces of current families recorded from HEK293 cells expressing WT (c), V400M (d), S241T (e), F1449V (f), VM/ST double mutant (g) and VM/FV double mutant (h) channels. Figure 2: Mutant cycle analysis of voltage dependence of activation of Na V 1.7 mutations. ( a ) Voltage dependence of activation curves of Na V 1.7 WT, V400M, S241T, and V400M/S214T (VM/ST) double mutant channels. Curves were Boltzmann fits of the data. ( b ) Voltage dependence of activation curves of Na V 1.7 WT, V400M, F1449V and V400M/F1449V (VM/FV) double mutant channels. ( c – h ) Representative traces of current families recorded from HEK293 cells expressing WT ( c ), V400M ( d ), S241T ( e ), F1449V ( f ), VM/ST double mutant ( g ) and VM/FV double mutant ( h ) channels. Full size image To quantitatively assess these effects, the energy change on channel activation caused by a single or double mutation was calculated. For each single or double mutation, V 1/2 and Z were used to determine free energy of activation (Δ G °). The change in free energy of mutants relative to the WT channel was designated as (ΔΔ G °) and coupling free energy (magnitude of non-additivity) was (∑Δ G °). Designation and calculation of (ΔΔ G °) and (∑Δ G °) are described in Methods. Based on previous studies [23] , [24] , [25] , [26] , [27] , [28] , we set the following standard: if |∑Δ G °|>1 kcal mol −1 , we accepted the two mutations as coupled (non-additive); whereas if |∑Δ G °|<1 kcal mol −1 , we accepted the two mutations as independent (additive). We calculated ∑Δ G ° for all mutation pairs and found that for the V400M:S241T mutation pair, ∑Δ G °=2.32 kcal mol −1 , and for V400M:F1449V mutation pair, the ∑Δ G °=−0.38 kcal mol −1 ( Supplementary Table S1 ). These data are in good agreement with the fitted curves, and strongly suggest that V400M and S241T are energetically coupled, whereas V400M and F1449V are energetically independent during channel activation. CBZ depolarizes S241T mutant channel activation Structural modelling showed atomic proximity between V400 and S241, and mutant cycle analysis demonstrated that S241T is energetically coupled with V400M during activation. Pretreatment of cells with a therapeutic concentration of CBZ (30 μM) is known to depolarize activation of V400M but not WT channels [9] . Although residues within S4–S5 linkers of sodium channels have not been implicated in forming the local anaesthetic-binding site [29] , we hypothesized that atomic proximity and energetic coupling of V400M and S241T might be paralleled by pharmacological coupling so that they might share pharmacoresponsiveness to CBZ. To test this hypothesis, the effect of CBZ (30 μM) pretreatment, initiated 30 min before recording [9] , on each mutant’s activation was measured in HEK293 cells expressing S241T or F1449V mutant channels. Representative recordings are shown in Fig. 3a–d . Notably, CBZ treatment caused a significant depolarizing shift in the V 1/2 of voltage dependence of activation of S241T mutant channels by 7.1 mV compared with dimethylsulphoxide (DMSO) treatment (DMSO: −37.6±1.0 mV, n =10; CBZ: −30.5±1.3 mV, n =13, P <0.01, Student’s t -test, Fig. 3e , Supplementary Table S2 ). In contrast, CBZ treatment of HEK293 cells expressing F1449V did not show a detectable effect on channel activation compared with DMSO treatment (activation V 1/2 for CBZ treatment: −27.1±1.5 mV, n =8; activation V 1/2 for DMSO treatment: −28.8±1.1 mV, n =9; P >0.05, Student’s t -test, Fig. 3f , Supplementary Table S2 ). 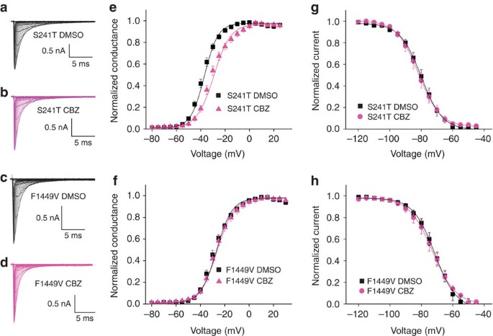Figure 3: Voltage dependence of activation and steady-state fast inactivation of S241T and F1449V mutant channels. (a–d) Representative traces of current families recorded from HEK293 cells expressing S241T mutant channel treated with DMSO (a), or with CBZ (b); F1449V mutant channel treated with DMSO (c), or with CBZ (d). (e) The averaged voltage dependence of activation of S241T mutant channel treated with DMSO or CBZ (30 μM) was plotted and fitted with Boltzmann equation. A depolarizing shift of activation of 7.1 mV was observed when S241T mutant channel was treated with CBZ (P<0.01, Student’st-test). (f) The averaged voltage dependence of activation of F1449V mutant channel treated with DMSO or CBZ was plotted and fitted with Boltzmann equation. No notable shift in activation curve of F1449V mutant channel was observed. (g–h) The voltage dependence of steady-state fast inactivation in response to 500 ms depolarizing potential for S241T (g) or F1449V (h) mutant channel treated with DMSO or CBZ was plotted and fitted with Boltzmann equation. No notable shift was observed. Figure 3: Voltage dependence of activation and steady-state fast inactivation of S241T and F1449V mutant channels. ( a – d ) Representative traces of current families recorded from HEK293 cells expressing S241T mutant channel treated with DMSO ( a ), or with CBZ ( b ); F1449V mutant channel treated with DMSO ( c ), or with CBZ ( d ). ( e ) The averaged voltage dependence of activation of S241T mutant channel treated with DMSO or CBZ (30 μM) was plotted and fitted with Boltzmann equation. A depolarizing shift of activation of 7.1 mV was observed when S241T mutant channel was treated with CBZ ( P <0.01, Student’s t -test). ( f ) The averaged voltage dependence of activation of F1449V mutant channel treated with DMSO or CBZ was plotted and fitted with Boltzmann equation. No notable shift in activation curve of F1449V mutant channel was observed. ( g – h ) The voltage dependence of steady-state fast inactivation in response to 500 ms depolarizing potential for S241T ( g ) or F1449V ( h ) mutant channel treated with DMSO or CBZ was plotted and fitted with Boltzmann equation. No notable shift was observed. Full size image Enhancement of steady-state fast inactivation (a hyperpolarizing shift of steady-state fast inactivation V 1/2 ) is a classic mechanism of action for CBZ [10] . However, for Na V 1.7, a therapeutic concentration of CBZ does not shift steady-state fast inactivation of WT channel [9] . To determine whether CBZ might have an effect on steady-state fast inactivation of S241T or F1449V mutant channels, HEK293 cells expressing S241T or F1449V mutant channels were treated with DMSO or CBZ (30 μM) as described earlier. Steady-state fast inactivation was assessed in response to a 500-ms depolarizing potential. This protocol demonstrated a steady-state fast inactivation V 1/2 for S241T of −79.9±1.7 mV ( n =6), and a steady-state fast inactivation V 1/2 for F1449 of −71.6±1.5 mV ( n =6) with DMSO treatment ( Supplementary Table S2 ), very close to the values found in our previous studies without any drug treatments [20] , [22] . CBZ (30 μM) did not significantly alter the V 1/2 for either S241T or F1449V mutant channels (−81.5±2.1 mV, n =6; −72.7±2.2 mV, n =8, respectively; P >0.05 compared with DMSO treatment, Student’s t -test, Fig. 3g ). Expression of S241T leads to DRG neuron hyperexcitability To study the effects of S241T mutant channel on nociceptor excitability, small (20–28 μm diameter) DRG neurons from postnatal day 1–5 rats were isolated and transfected with either human Na V 1.7 WT or S241T mutant channels. Excitability was assessed by current-clamp recording 2 days after transfection. Current threshold, the injection current required to produce a single all-or-none action potential, was determined by applying 200 ms depolarizing currents of increasing magnitude (5 pA increments). For the neuron transfected with WT channels shown in Fig. 4a , current injection smaller than 225 pA generated small, graded membrane potential depolarization, with the first all-or-none action potential elicited by current injection of 230 pA. In contrast, a neuron expressing the S241T mutant channel fired the first action potential in response to current injection of 60 pA ( Fig. 4b ). On average, expression of S241T mutant caused a significant ~2.7-fold reduction of action potential threshold (83.5±18.2 pA, n =20) compared with DRG neurons expressing WT channel (227.6±36.7 pA, n =19, P <0.01, Student’s t -test, Fig. 4c ). 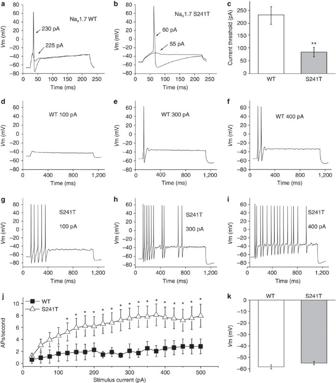Figure 4: Current-clamp analysis of DRG neurons expressing WT or S241T mutant channel. (a) Representative DRG neuron expressing NaV1.7 WT channel showed sub-threshold response to 225 pA current injection and subsequent action potential evoked by injection of 230 pA, which was the current threshold for this neuron. (b) Representative DRG neuron expressing NaV1.7-S241T mutant channel showed sub-threshold response to 55 pA current injection and subsequent action potential evoked by injection of 60 pA. (c) Comparison of current threshold for DRG neurons expressing WT and S241T mutant channels. Expression of S241T channel reduced current threshold significantly (**P<0.01, Student’st-test). Current threshold for WT: (227.6±36.7 pA,n=19); for S241T: (83.5±18.2 pA,n=20). (d–f) Responses of a representative DRG neuron expressing WT channel to 1-s-long depolarizing current steps at 100 (d), 300 (e) and 400 (f) pA current injection. (g–i) Responses of a representative DRG neuron expressing S241T mutant channel to 1-s-long depolarizing current steps at 100 (g), 300 (h) and 400 (i) pA current injection. The difference in responses is apparent across this range. (j) The averaged number of action potentials between DRG neurons expressing WT and S241T mutant channel was compared. The response of DRG neurons expressing WT channel to current injection was significantly different compared with DRG neurons expressing S241T mutant channel across a range (125–500 pA) of step current injections (*P<0.05, Mann–Whitney test). (k) Averaged resting membrane potentials for DRG neurons expressing WT or S241T mutant channel were not statistically different. Results are presented as mean±s.e.m. Figure 4: Current-clamp analysis of DRG neurons expressing WT or S241T mutant channel. ( a ) Representative DRG neuron expressing Na V 1.7 WT channel showed sub-threshold response to 225 pA current injection and subsequent action potential evoked by injection of 230 pA, which was the current threshold for this neuron. ( b ) Representative DRG neuron expressing Na V 1.7-S241T mutant channel showed sub-threshold response to 55 pA current injection and subsequent action potential evoked by injection of 60 pA. ( c ) Comparison of current threshold for DRG neurons expressing WT and S241T mutant channels. Expression of S241T channel reduced current threshold significantly (** P <0.01, Student’s t -test). Current threshold for WT: (227.6±36.7 pA, n =19); for S241T: (83.5±18.2 pA, n =20). ( d – f ) Responses of a representative DRG neuron expressing WT channel to 1-s-long depolarizing current steps at 100 ( d ), 300 ( e ) and 400 ( f ) pA current injection. ( g – i ) Responses of a representative DRG neuron expressing S241T mutant channel to 1-s-long depolarizing current steps at 100 ( g ), 300 ( h ) and 400 ( i ) pA current injection. The difference in responses is apparent across this range. ( j ) The averaged number of action potentials between DRG neurons expressing WT and S241T mutant channel was compared. The response of DRG neurons expressing WT channel to current injection was significantly different compared with DRG neurons expressing S241T mutant channel across a range (125–500 pA) of step current injections (* P <0.05, Mann–Whitney test). ( k ) Averaged resting membrane potentials for DRG neurons expressing WT or S241T mutant channel were not statistically different. Results are presented as mean±s.e.m. Full size image The firing frequency of DRG neurons was also assessed by a series of 1-s current injections from 25 to 500 pA in 25-pA increments. For DRG neurons expressing WT channel, no action potentials or only a single action potential was elicited in response to depolarizing current injection, with an occasional second spike in response to stronger stimuli ( Fig. 4d–f ). In contrast, DRG neurons expressing S241T fired repetitively in response to low and high current injections ( Fig. 4g–i ). To compare firing frequency of DRG neurons expressing WT or S241T channels, the number of spikes elicited by 1-s current injection at various stimulus intensities was averaged ( Fig. 4j ). DRG neurons expressing S241T mutant channel fired significantly more spikes than DRG neurons expressing WT channel at all stimulus intensities ≥125 pA ( Fig. 4j , P <0.05, Mann–Whitney test). Resting membrane potential (RMP) is known to affect DRG neuron excitability [30] . We therefore also assessed RMP of DRG neurons expressing WT or S241T mutant channels but did not observe a significant difference in RMPs ( Fig. 4k ). Taken together, these data show that expression of S241T mutant channels induces DRG neuron hyperexcitability. CBZ normalizes excitability of DRG neurons expressing S241T To test the prediction from our structural modelling and mutant cycle analysis, we assessed the effect of CBZ on hyperexcitability of DRG neurons expressing S241T or F1449V mutant channels using current-clamp recording. DRG neurons were treated with either DMSO or CBZ (30 μM) initiated 30 min before recording as mentioned above. Current threshold was assessed first: the response of a representative neuron expressing S241T treated with DMSO is shown in Fig. 5a . Current threshold for this neuron was 75 pA. In contrast, current threshold of a representative neuron expressing S241T treated with CBZ is shown in Fig. 5b . Current threshold for this neuron is 170 pA. On average, CBZ treatment resulted in a significant ~two fold increase in current threshold for DRG neurons expressing S241T mutant channel (CBZ treatment: 162.7±24.4 pA, n =28; DMSO treatment: 90.4±13.2 pA, n =27, P <0.01, Student’s t -test; Fig. 5c ), indicating that CBZ treatment is likely to attenuate the excitability of DRG neurons expressing S241T mutant channel. 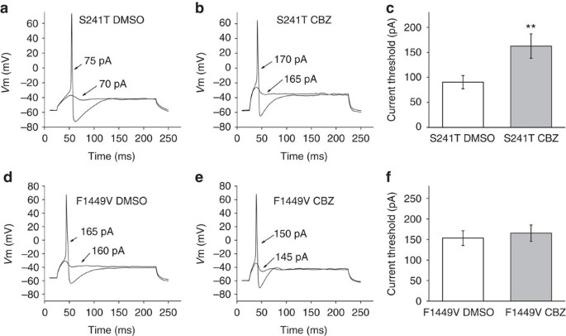Figure 5: Current thresholds of CBZ- or DMSO-treated DRG neurons expressing S241T or F1449V mutant channels. (a,b) Sub- and supra-threshold responses of representative DRG neurons expressing S241T mutant channel treated with DMSO (a) or 30 μM CBZ (b) are shown. (c) Comparison of current threshold for DRG neurons expressing S241T mutant channel treated with DMSO or 30 μM CBZ. CBZ treatment increased the current threshold significantly (**P<0.01, Student’st-test). Current threshold for DMSO-treated DRG neurons: 90.4±13.2 pA (n=27); for CBZ-treated DRG neurons: 162.7±24.4 pA (n=28). (d,e) Sub- and supra-threshold responses of DRG neurons expressing F1449V mutant channel treated with DMSO (d) or 30 μM CBZ (e) are shown. (f) Comparison of current threshold for DRG neurons expressing F1449V mutant channel with the treatment of DMSO (153.5±17.9 pA,n=29) or 30 μM CBZ (165.5±19.7 pA,n=28). No significant difference was found (P>0.05, Student’st-test). Results are presented as mean±s.e.m. Figure 5: Current thresholds of CBZ- or DMSO-treated DRG neurons expressing S241T or F1449V mutant channels. ( a,b ) Sub- and supra-threshold responses of representative DRG neurons expressing S241T mutant channel treated with DMSO ( a ) or 30 μM CBZ ( b ) are shown. ( c ) Comparison of current threshold for DRG neurons expressing S241T mutant channel treated with DMSO or 30 μM CBZ. CBZ treatment increased the current threshold significantly (** P <0.01, Student’s t -test). Current threshold for DMSO-treated DRG neurons: 90.4±13.2 pA ( n =27); for CBZ-treated DRG neurons: 162.7±24.4 pA ( n =28). ( d , e ) Sub- and supra-threshold responses of DRG neurons expressing F1449V mutant channel treated with DMSO ( d ) or 30 μM CBZ ( e ) are shown. ( f ) Comparison of current threshold for DRG neurons expressing F1449V mutant channel with the treatment of DMSO (153.5±17.9 pA, n =29) or 30 μM CBZ (165.5±19.7 pA, n =28). No significant difference was found ( P >0.05, Student’s t -test). Results are presented as mean±s.e.m. Full size image Our previous studies demonstrated that expression of F1449V mutant channel in DRG neurons reduces the current threshold and increases the firing frequency in response to sustained depolarizing stimuli [21] . As CBZ did not produce a depolarizing shift in F1449V mutant channel activation curve ( Fig. 3f ), we hypothesized that CBZ would not normalize firing properties of DRG neurons expressing F1449V mutant channel. Again, we assessed the current threshold first: as illustrated in Fig. 5d , current threshold of DRG neurons expressing F1449V mutant channels was similar between CBZ and DMSO treatments. For the population of neurons in these experiments, no significant difference was found for current threshold (DMSO, 153.5±17.9 pA, n =29; CBZ, 165.5±19.7 pA, n =28, P >0.05, Student’s t -test, Fig. 5f ). We further tested the effect of CBZ treatment on the firing frequency of DRG neurons expressing either the S241T or F1449V mutant channels. Robust repetitive firing was seen for neurons expressing S241T mutant channel treated with DMSO ( Fig. 6a–c ). In contrast, pretreatment with CBZ dramatically reduced the number of action potentials in DRG neurons expressing S241T mutant channel ( Fig. 6d–f ), with a statistically significant reduction of firing frequency at all stimulus intensities ≥100 pA ( P <0.05, Mann–Whitney test, Fig. 6g ). This effect was not confounded by changes in RMPs, as CBZ did not affect RMPs of DRG neurons expressing mutant channels ( Figs 6h and 7h ). Taken together, our data demonstrate that CBZ attenuates the hyperexcitability of DRG neurons expressing S241T mutant channel. 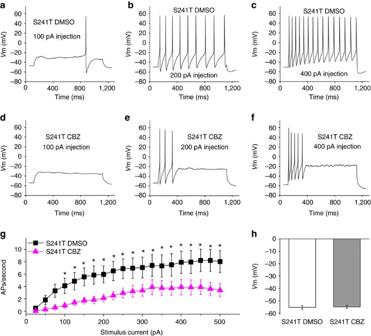Figure 6: Firing frequencies and membrane potentials of CBZ- or DMSO-treated DRG neurons expressing S241T. (a–c) Responses of a representative DRG neuron expressing S241T mutant channel treated with DMSO to 1 s long depolarization current steps at 100 (a), 200 (b) and 400 (c) pA current injection. (d–f) Similar recordings from a representative DRG neuron expressing S241T mutant channel treated with 30 μM CBZ at 100 (d), 200 (e), and 400 (f) pA current injection. (g) Averaged response for DRG neurons expressing S241T mutant channel treated with DMSO (n=27) or CBZ (n=28) are summarized. CBZ statistically reduced firing frequency starting from 100 pA current injection (*P<0.05, Mann–Whitney test). (h) Averaged RMP between DRG neurons expressing S241T mutant channel treated with DMSO or CBZ were not statistically different (DMSO: −55.3±1.4 mV,n=27; CBZ: −54.9±1.3 mV,n=28,P>0.05, Student’st-test). Results are presented as mean±s.e.m. Figure 6: Firing frequencies and membrane potentials of CBZ- or DMSO-treated DRG neurons expressing S241T. ( a – c ) Responses of a representative DRG neuron expressing S241T mutant channel treated with DMSO to 1 s long depolarization current steps at 100 ( a ), 200 ( b ) and 400 ( c ) pA current injection. ( d – f ) Similar recordings from a representative DRG neuron expressing S241T mutant channel treated with 30 μM CBZ at 100 ( d ), 200 ( e ), and 400 ( f ) pA current injection. ( g ) Averaged response for DRG neurons expressing S241T mutant channel treated with DMSO ( n =27) or CBZ ( n =28) are summarized. CBZ statistically reduced firing frequency starting from 100 pA current injection (* P <0.05, Mann–Whitney test). ( h ) Averaged RMP between DRG neurons expressing S241T mutant channel treated with DMSO or CBZ were not statistically different (DMSO: −55.3±1.4 mV, n =27; CBZ: −54.9±1.3 mV, n =28, P >0.05, Student’s t -test). Results are presented as mean±s.e.m. 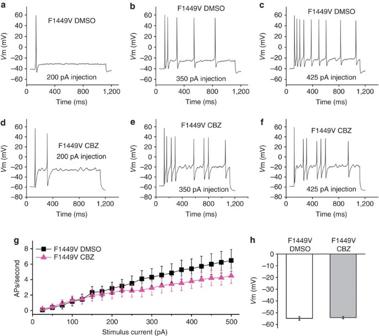Figure 7: Firing frequencies and membrane potentials of CBZ- or DMSO-treated DRG neurons expressing F1449V. (a–c) Responses of a representative DRG neurons expressing F1449V mutant channel treated with DMSO to 1-s-long depolarization current steps at 200 (a), 350 (b) and 425 (c) pA current injection. (d–f) Similar recordings from a representative DRG neuron expressing F1449V mutant channel treated with CBZ at 200 (d), 350 (e) and 425 (f) pA current injection. (g) Averaged firing frequencies for DRG neurons expressing F1449V mutant channel treated with DMSO (n=29) or CBZ (n=28) were compared and no statistical difference was found across the entire range (P>0.05, Mann–Whitney test). (h) Averaged RMPs between DRG neurons expressing F1449V mutant channel treated with DMSO or CBZ were not statistically different (DMSO: −54.8±1.5 mV,n=29; CBZ: −54.1±1.0 mV,n=28,P>0.05, Student’st-test). Results are presented as mean±s.e.m. Full size image Figure 7: Firing frequencies and membrane potentials of CBZ- or DMSO-treated DRG neurons expressing F1449V. ( a – c ) Responses of a representative DRG neurons expressing F1449V mutant channel treated with DMSO to 1-s-long depolarization current steps at 200 ( a ), 350 ( b ) and 425 ( c ) pA current injection. ( d – f ) Similar recordings from a representative DRG neuron expressing F1449V mutant channel treated with CBZ at 200 ( d ), 350 ( e ) and 425 ( f ) pA current injection. ( g ) Averaged firing frequencies for DRG neurons expressing F1449V mutant channel treated with DMSO ( n =29) or CBZ ( n =28) were compared and no statistical difference was found across the entire range ( P >0.05, Mann–Whitney test). ( h ) Averaged RMPs between DRG neurons expressing F1449V mutant channel treated with DMSO or CBZ were not statistically different (DMSO: −54.8±1.5 mV, n =29; CBZ: −54.1±1.0 mV, n =28, P >0.05, Student’s t -test). Results are presented as mean±s.e.m. Full size image In contrast, CBZ did not attenuate the abnormal repetitive firing of DRG neurons expressing F1449V mutant channel. Repetitive firing was observed for neurons expressing F1449V mutant channel treated with DMSO ( Fig. 7a–c ) as well as treated with CBZ ( Fig. 7d–f ). Across a range of current injections, the firing frequency for CBZ- and DMSO-treated neurons was comparable in response to current injection ≤200 pA ( Fig. 7g ). Although firing frequency started to diverge with stronger injection, the effect of CBZ did not reach statistical significance even at current injection of 500 pA ( Fig. 7g ). Together with our results on V400M and S241T mutant channels, these data suggest that the effect of CBZ is mutant specific and agrees well with our predication from structural modelling and mutant cycle analysis. Using structural modelling, based upon the recently solved crystal structure of a bacterial voltage-gated sodium channel [13] , we report that S241 within the DI/S4–S5 linker, while 159 amino acids distant from V400 in the channel peptide, is located close to V400 in the folded structure of the human Na V 1.7 sodium channel. Using mutant cycle analysis, we have demonstrated that Na V 1.7-V400M and -S241T mutant channels are energetically coupled during channel activation, suggesting that they contribute to the same feature of activation. As V400M mutation responds favourably to CBZ by shifting activation of V400M [9] , we reasoned that energetic coupling of V400M and S241T during channel activation might be paralleled by pharmacological coupling. Using voltage-clamp recording, we found that a therapeutic concentration of CBZ indeed normalizes the activation of S241T mutant channel. Moreover, we further show that this normalization of activation is accompanied by increased current threshold and reduced firing frequency of DRG neurons expressing S241T mutant channel. In contrast, V400M and F1449V mutants were not energetically coupled, and CBZ had no detectable effect on activation of F1449V or on the firing properties of DRG neurons expressing F1449V mutant channel. Human and rodent studies have demonstrated that the Na V 1.7 channel is essential for pain signalling and have validated this channel as a promising drug target for the development of novel pain therapeutics [4] . Structural and functional studies of Na V 1.7 mutant channels may provide insight into understanding mechanistic features of channel gating and its interaction with drugs. Previous studies of sodium channel structure and function were largely based on information obtained from the crystal structure of potassium channels [22] , [25] , [31] . Availability of the crystal structure of a bacterial voltage-gated sodium channel NavAb [13] permitted construction of a more realistic mammalian voltage-gated sodium channel model. It is worth noting that bacterial Na V channels are four-fold symmetric, assembled from identical subunits, whereas mammalian Na V channels have four non-identical domains encoded by a single protein. Alignment of NavAb and the four transmembrane domains of the Na V 1.7 channel is shown in Supplementary Table S3 and superposition of the transmembrane domains of Na V 1.7 with NavAb is shown in Fig. 8 . Despite the difference outlined above, the bacterial Na V channel is the closest template for studying mammalian Na V channel. Additionally, recent enhancements to I-TASSER [17] , a protein prediction package that has been successfully used to predict structure of many proteins including potassium channels for functional studies [32] , [33] , have provided improved predictions of membrane-bound proteins structure [15] , [34] . This method is not a simple homology modelling tool because the threading alignments from templates have been broken into pieces, which are used to reassemble the global structure of the membrane domains under the guide of a composite physics- and knowledge-based force field. As a result, it has been systematically demonstrated in community-wide CASP experiments that GPCR-ITASSER models can be significantly closer to the target structure than the homologous modelling [35] . Taking advantage of these new developments, we constructed a structural model for the human Na V 1.7 channel and used it in this study to investigate the participation of different residues in channel activation, and to make predictions about drug–channel interaction. 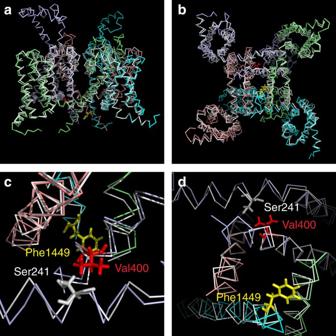Figure 8: Alignment of NaV1.7 structural model with NavAb structure. (a) Intra-membrane view of structural model of NaV1.7 channel transmembrane domains aligned with NavAb structure (3RVY). NaV1.7 Domain I, lightblue; Domain II, salmon; Domain III, cyan; Domain IV, lime. NavAb, white. (b) Cytosolic view of the structural model of NaV1.7 channel transmembrane domains aligned with NavAb structure. (c) Close-up intra-membrane side view of the area containing S241 (grey), V400 (red) and F1449 (yellow) residues. (d) Close-up cytosolic view of the area containing S241, V400 and F1449 residues. Figure 8: Alignment of Na V 1.7 structural model with NavAb structure. ( a ) Intra-membrane view of structural model of Na V 1.7 channel transmembrane domains aligned with NavAb structure (3RVY). Na V 1.7 Domain I, lightblue; Domain II, salmon; Domain III, cyan; Domain IV, lime. NavAb, white. ( b ) Cytosolic view of the structural model of Na V 1.7 channel transmembrane domains aligned with NavAb structure. ( c ) Close-up intra-membrane side view of the area containing S241 (grey), V400 (red) and F1449 (yellow) residues. ( d ) Close-up cytosolic view of the area containing S241, V400 and F1449 residues. Full size image We used thermodynamic mutant cycle analysis, a well-established tool, to quantitatively assess the energetic independence or coupling of two mutations in affecting channel activation. Mutant cycle analysis has been used to understand transition of pore elements during potassium channel gating [23] , interactions between ion channels and toxins [24] , [28] and identification of ion-pair-forming residues of the voltage-sensor domain in a bacterial sodium channel (NaChBac) during voltage-gated activation [25] , [26] , [27] . We show here that mutant cycle analysis can be used to test the hypothesis that different pathogenic IEM mutations (S241T, V400M and F1449V), all of which cause a hyperpolarizing shift of channel activation, participate in different steps of channel gating and have distinct pharmacoresponsiveness. More importantly, this analysis allowed us to predict that S241T mutant channel may interact with CBZ in a similar fashion as V400M mutant channel owing to their energetic coupling for channel activation. Our structural model revealed that the V400 side chain points towards the DI/S4–S5 linker and is atomically close to and facing the S241 residue located in this linker, suggesting that mutations of these two residues might affect the same step in channel activation. The interaction between S4–S5 linker and S6 during channel gating has been suggested in voltage-gated K + (K V ) channel [36] , [37] , [38] . More recently, an all-atom molecular dynamics study of K V channel gating mechanism has extended these findings by showing that channel activation imposes a pulling force on S4–S5 linker, which perturbs the interaction between S4–S5 linker and S6, leading to channel opening [39] . Coupling of pore-forming helix to voltage sensors is also seen in Na V channels [40] , [41] , most likely through S4–S5 linker [42] . A residue at the beginning of the S4–S5 linker is likely to form an interacting pair with residue at the tail end of the S6 helix [42] , further supporting the potential interaction of S4–S5 linker and S6 helix. On the other hand, F1449V may affect different steps in activation: the Na V 1.7 structural model places F1449 at the cytoplasmic tip of the S6 helix, suggesting that F1449 contributes to a hydrophobic ring at the cytoplasmic vestibule of the pore, consists of aromatic residues at equivalent positions in the S6 from four domains, acting as the activation gate of the channel. Taken together, our results suggest that V400M or S241T mutation may disrupt the tight packing of S4–S5 linker with S6 pore-forming helix, affecting channel activation; whereas the F1449V mutation may disrupt the hydrophobic ring and destabilize the channel pre-open state, hyperpolarizing activation via a different structural action [21] , [22] . Mutational analysis and functional studies have identified residues within S6 segments of domains III and IV to be important in forming drug-binding site(s) for local anaesthetic and antiepileptic drugs, including CBZ (see [43] , [44] , [45] for review). The binding of a few sodium channel blockers (for example, local anaesthetic drugs, anticonvulsant drugs) to the pore of voltage-gated sodium channels has been studied using structural modeling [29] , [46] . CBZ has been shown to interact with three key residues of Na V 1.2 channel (Leu1465 of DIII-S6, Phe1764 of DIV-S6 and Tyr1771 of DIV-S6) [29] . In addition, N434, located near the middle of the DI/S6 helix, is also important for drug binding of Na V 1.4 ( [47] ). IEM mutation N395K of Na V 1.7 channel, which corresponds to N434 in Na V 1.4, is suggested to be located within the local anaesthetic-binding site of Na V 1.7. N395K mutation has been shown to depolarize activation of Na V 1.7 as well as significantly reduce use-dependent inhibition by lidocaine [11] . In addition, it has been found that the binding of local anaesthetics (for example, lidocaine) to Na V channel may lead to allosteric coupling of the binding site(s) of pore-forming helix to voltage sensors, especially in domain III and IV [48] . It is further suggested that S4–S5 linker and the intracellular end of S5 and S6 may be critical in coupling S6 helix to voltage-sensor movement in the presence of local anaesthetics [49] . These results imply that the effects of CBZ on Na V 1.7-S241T and -V400M mutant channels are not likely to be attributable to direct effects of these mutations on the drug-binding site(s). Alternatively, our data may be interpreted as suggesting a role for CBZ as a chemical chaperone for S241T and V400M mutant channels, rather than as a channel blocker. According to this hypothesis, CBZ–channel interaction may lead to stabilization of the S241T and V400M mutant channel in a WT-like conformation, and cause a depolarizing shift in activation, a biophysical change that contributes to attenuation of hyperexcitability of DRG neurons expressing mutant channels. In summary, our results demonstrate that structural modelling and mutant cycle analysis can reveal the effect of sodium channel mutations on channel gating, and predict the responses of sodium channel mutations to a pharmacotherapeutic agent. We suggest that a similar approach, initially screening channels of interest for amino-acid variants that enhance pharmacoresponsiveness to existing agents and then using these variants as ‘seeds’ for further identification of other variants that enhance pharmacosensitivity, may permit identification of genomically defined subgroups of the population that are pharmacoresponsive. Structural modelling Mammalian Na V 1.7 sodium channel is made up of four transmembrane domains, named I, II, III, IV linked by cytoplasmic loops. The transmembrane helix structural model of human Na V 1.7 sodium channel was constructed in two steps. First, each of the four transmembrane domains was modelled separately using an advanced membrane-bound protein prediction algorithm GPCR-ITASSER [16] , [50] , [51] . Then, the whole channel model was built by structurally aligning four individual domain models to a global structural template of the recently solved bacterial sodium channel. The GPCR-ITASSER algorithm is an advanced algorithm for transmembrane helical structure modelling. The program first uses a multiple threading procedure LOMETS [14] to identify the putative-related template structures in the PDB. The structural fragments (mainly α-helices) are then excised from the threading templates and assembled into full-length models by replica-exchange Monte Carlo simulations. In addition to the inherent I-TASSER force field, five transmembrane-protein-specific energy terms were also used to describe the interactions between transmembrane domain and membrane. (1) Membrane-repulsive energy is introduced for reducing the clash between intra- and extracellular domain and bilayer membrane. (2) Extracellular hydrophilic interactions for the hydrophilic interactions for residues inside and outside membrane. (3) Hydrophobic moment energy for the hydrophobic interaction between transmembrane helix and membrane. (4) Aromatic interactions for enhancing the specific interactions between aromatic–aromatic residues. (5) Cation–π interactions for specific non-covalent-binding propensities between TM helices. Finally, models of the lowest free energy are identified by clustering the simulation trajectories using SPICER [52] , and are refined at the atomic level by a fragment-guided dynamic simulation program FG-MD [50] . We assembled the four transmembrane domains models in a clockwise order viewed from extracellular side as suggested by previous literature [53] , [54] . Each single domain model was aligned to the corresponding domain of the recently solved bacterial sodium channel by the structural alignment algorithm TM-align [55] . The resultant four domain complete structural model was refined again by FG-MD [50] to accommodate inter-domain steric clashes and improve the model quality. Plasmid preparation and HEK293 cell transfection TTX-resistant human Na V 1.7 wild-type (WT) channel (hNa V 1.7r) was created based on the hNa V 1.7 (GenBank accession codes: NM_002977.3 (mRNA); NP_002968.1 (protein). All other tested mutations were constructed on hNa V 1.7r background using Quick Change XL site-directed mutagenesis kit (Stratagene, La Jolla, CA, USA). WT or the mutant channels were transfected into HEK293 cells together with human β-1 and β-2 subunit [56] using Lipofectamine reagent (Invitrogen, Carlsbad, CA, USA). HEK293 cells were maintained in 1:1 Dulbecco’s modified Eagle’s media (DMEM)/F12 supplemented with 10% fetal bovine serum (FBS, Hyclone) in a humidified 5% CO 2 incubator at 37 °C. HEK293 cells were seeded onto poly-l-lysine-coated glass coverslips (BD Biosciences, San Jose, CA, USA) in a 24-well plate 1 day before transfection. Recording was performed 1 day after transfection. Voltage-clamp recording of sodium channel in HEK cells Whole-cell voltage-clamp recordings were performed using the following solutions: the extracellular solution contained the following (in mM): 140 NaCl, 3 KCl, 1 MgCl 2 , 1 CaCl 2 , 20 Dextrose and 10 HEPES, pH=7.3 with NaOH (320 mOsm adjusted with dextrose). The pipette solution contained the following (in mM): 140 Cs-Fluoride, 10 NaCl, 1.1 EGTA, 10 HEPES, 20 Dextrose, pH=7.3 with CsOH (310 mOsm adjusted with dextrose). Patch pipettes had a resistance of 1–2 mΩ when filled with pipette solution. After achieving whole-cell recording configuration, the pipette and cell capacitance were manually minimized using the Axopatch 200B (Molecular Devices) compensation circuitry. Series resistance and prediction compensation (80–90%) was applied to reduce voltage errors. The recorded currents were digitized using pClamp software and a Digidata 1440A interface (Molecular Devices) at a rate of 50 kHz after passing through a low-pass Bessel filter setting of 10 kHz. Linear leak and residual capacitance artifacts were subtracted out using a P/N method provided with the Clampex software. Recording was initiated after a 5-min equilibration period after breaking in whole-cell configuration. CBZ was purchased from Sigma, dissolved in DMSO. For CBZ experiments, cells were treated with either CBZ (30 μM) or DMSO in incomplete medium without FBS for 30 min before recording and the CBZ or DMSO was maintained in the bath solution during the recording as described previously [9] . Data analysis was performed using Clampfit (Molecular Devices) and Origin (Microcal Software). To generate activation curves, cells were held at −120 mV and stepped to potentials of −80 to +40 mV in 5-mV increments for 100 ms. Peak inward currents were automatically extracted by Origin and fitted with BoltzIV function to determine the voltage at half activation ( V 1/2 ), activation curve slope at half activation ( Z ) and reversal potential ( E Na ) for each recording. Conductance was calculated as G = I /( V m− E Na ) and normalized by the maximum conductance value and fit with Boltzmann equation. To generate steady-state fast-inactivation curves, cells were stepped to inactivating potentials from −120 to −40 mV for 500 ms followed by a 40-ms step to −10 mV as described previously [21] , [57] . Peak inward currents obtained from steady-state fast inactivation were normalized by maximum current amplitude and fitted with a Boltzmann equation. Mutant cycle analysis Double mutations (VM/ST and VM/FV) were created using site-directed mutagenesis. A total of six constructs (WT, V400M, S241T, F1449V, VM/ST, VM/FV) were expressed in HEK293 cells separately for patch-clamp analysis. The voltage dependence of activation for these mutations was analysed and a G – V curve was generated and fitted with Boltzmann equation to obtain V 1/2 and Z . Using V 1/2 and Z , the free energy to switch the channel from closed to the open state was calculated as Δ G ° (C→O) (kcal/mol)=− FZV 1/2 . The additional free energy required for the mutant channel to open relative to the WT channel was calculated as ΔΔ G °=Δ( FZV 1/2 )=− F ( Z mut V 1/2mut − Z wt V 1/2wt ). Magnitude of non-additivity (or the non-additive coupling free energy) was calculated as ΣΔ G °=ΔΔ( FZV 1/2 )=− F [( Z wt V 1/2wt − Z mut1 V 1/2mut1 )−( Z mut2 V 1/2mut2 − Z mut1 , mut2 V 1/2 mut1,mut2 )] (refs 23 , 24 , 25 , 26 , 27 , 28 ). Isolation and transfection of DRG neurons DRG of Sprague-Dawley rat pups (postnatal day 1–5) were isolated and cultured as described previously [58] , [59] . Dissected ganglia were placed in ice-cold oxygenated complete saline solution (CSS), which contained the following (in mM): 137 NaCl, 5.3 KCl, 1 MgCl 2 , 25 sorbitol, 3 CaCl 2 and 10 HEPES, pH 7.2. DRGs were then transferred to oxygenated 37 °C CSS solution containing 1.5 mg ml −1 collagenase A (Roche Applied Science) and 0.6 mM EDTA and incubated with gentle agitation at 37 °C for 20 min. This solution was exchanged with oxygenated, 37 °C CSS solution containing 1.5 mg ml −1 collagenase D (Roche Applied Science), 0.6 mM EDTA and 30 U ml −1 papain (Worthington Biochemicals) and incubated with gentle agitation at 37 °C for 20 min. The solution was then aspirated and ganglia were triturated in DRG media: DMEM/F12 (1:1) with 100 μ ml −1 penicillin, 0.1 mg ml −1 streptomycin (Invitrogen), and 10% FBS, which contained 1.5 mg ml −1 bovine serum albumin (Sigma-Aldrich) and 1.5 mg ml −1 trypsin inhibitor (Roche Applied Science). WT, S241T or F1449V mutant channels were transiently transfected into the DRG neurons, respectively, along with enhanced green fluorescent protein (GFP), by electroporation with a Nucleofector II (Amaxa) system using basic Neuron SCN Nucleofector and program ‘SCN basic program 6’. The ratio of sodium channel to GFP constructs was 10:1. Transfected neurons were allowed to recover for 5 min at 37 °C in 0.5 ml of Ca ++ -free DMEM. The cell suspension was then diluted with DRG media containing 1.5 mg ml −1 bovine serum albumin and 1.5 mg ml −1 trypsin inhibitor, 80 μl mixture was placed on 12 mm circular poly-d-lysine/laminin-precoated coverslips (BD biosciences), and the cells were incubated at 37 °C in 5% CO 2 for 30 min. DRG media (1 ml per well), supplemented with 50 ng ml −1 each of mouse NGF (Alomone Labs) and glial cell line-derived neurotrophic factor (GDNF, Peprotec), was then added to cells. Cells were maintained at 37 °C in a 5% CO 2 incubator for further experiments. Current-clamp recording in transfected DRG neurons Whole-cell configuration was obtained in voltage-clamp mode before starting current-clamp recording. The pipette solution contained (in mM): 140 KCl, 0.5 EGTA, 3 Mg-ATP, 5 HEPES, 30 dextrose, pH=7.3 with KOH (310 mOsmol l −1 ). The extracellular bath solution contained (in mM): 140 NaCl, 3 KCl, 2 MgCl 2 , 2 CaCl 2 , 15 dextrose, 10 HEPES, pH=7.3 with NaOH (315 mOsmol l −1 ). Recording was performed on transfected nociceptive neurons, based on morphology with criteria of small diameter (20–28 μm) and round cell bodies, which also exhibited GFP fluorescence. All recordings were performed 2 days after transfection. For CBZ experiments, neurons were treated with either CBZ (30 μM) or DMSO as described above. RMP and seal stability for each neuron were evaluated during a 30-s-long period. Current threshold for action potential generation was determined by a series of 200 ms depolarizing currents in 5-pA increments. Repetitive firing frequency was examined using a series of 1-s current steps from 25 to 500 pA in 25-pA increments. The interval between stimuli was 10 s. For firing frequency measurement, spikes with overshoot beyond 0 mV were counted as action potentials. Data analysis Data were analysed with Clampfit 9.2 (Molecular Devices) and OriginPro 8.5 (Microcal Software). For statistical analysis, if samples obeyed a normal distribution, Student’s t -test was used. Non-parametric Mann–Whitney test was used when samples failed the normality test. Data was presented as means±s.e.m. Statistical significance was accepted when P <0.05. How to cite this article: Yang, Y. et al. Structural modeling and mutant cycle analysis predict pharmacoresponsiveness of a Na v 1.7 mutant channel. Nat. Commun. 3:1186 doi: 10.1038/ncomms2184 (2012).